Mechanism of 150-cavity formation in influenza neuraminidase The recently discovered 150-cavity in the active site of group-1 influenza A neuraminidase (NA) proteins provides a target for rational structure-based drug development to counter the increasing frequency of antiviral resistance in influenza. Surprisingly, the 2009 H1N1 pandemic virus (09N1) neuramidase was crystalized without the 150-cavity characteristic of group-1 NAs. Here we demonstrate, through a total sum of 1.6 μs of biophysical simulations, that 09N1 NA exists in solution preferentially with an open 150-cavity. Comparison with simulations using avian N1, human N2 and 09N1 with a I149V mutation and an extensive bioinformatics analysis suggests that the conservation of a key salt bridge is crucial in the stabilization of the 150-cavity across both subtypes. This result provides an atomic-level structural understanding of the recent finding that antiviral compounds designed to take advantage of contacts in the 150-cavity can inactivate both 2009 H1N1 pandemic and avian H5N1 viruses. Understanding the structural dynamics of the influenza glycoproteins has been a long-standing goal because of their direct impact on public health. The two major influenza glycoproteins, hemagglutinin (HA) and neuraminidase (NA), control entry and exit of the viral particles from the host cell, respectively. HA binds to sialic acid surface receptors on the host cell, whereas NA cleaves the terminal sialic acid receptor linkage, facilitating viral shedding. The nine NA alleles have been divided into two groups based on phylogenetic analysis (group-1: N1, N4, N5, N8; group-2: N2, N3, N6, N7, N9) [1] . During the last century, influenza viruses carrying N1 (H1N1) or N2 (H2N2, H3N2) alleles have circulated in humans, first as pandemic strains and then, after subsequent adaptation to humans, as seasonal epidemic strains. Thus, a better understanding of the structural dynamics of N1 and N2 is particularly relevant for antiviral design. Oseltamivir (Tamiflu) and zanamivir (Relenza), which target the NA, are currently the only antivirals approved by the FDA for the prophylaxis and treatment of influenza. These drugs, developed against available group-2 NA structures, represent some of the first successful rational structure-based drug development efforts [2] . The crystal structures of group-1 NAs revealed a never-before-seen 150-cavity adjacent to the sialic-acid-binding site [1] . It has been hypothesized, and very recently shown [3] , that targeting the 150-cavity may allow the development of new antivirals with increased specificity and potency against group-1 enzymes. The increasing frequency of oseltamivir resistance in pre-2009 seasonal H1N1 viruses [4] and the occasional observation of oseltamivir resistance among 2009 H1N1 pandemic viruses motivates new antiviral development. Having additional antivirals in our treatment arsenal would be advantageous, and potentially critical, if a highly virulent strain, for example, H5N1, evolved the ability to undergo rapid transmission among humans or if the already highly transmissible 2009 H1N1 pandemic virus was to evolve resistance to existing antiviral drugs. Recently, it was revealed that the structure of the 2009 pandemic H1N1 NA lacked a 150-cavity, despite being a group-1 NA [5] . This surprising finding suggested that the 2009 pandemic N1 protein was structurally more similar to the group-2 NAs than to the group-1 NAs. Based on alignments of sequences representing all available NA crystal structures, highly conserved residues in the 150-loop and the 430-loop (residues 147–152 and 429–433, respectively, in N2 numbering) were hypothesized to functionally determine the structure of the 150-cavity [5] . In particular, I149 was found to be common between the 2009 pandemic N1 and group-2 NAs, whereas V149 was conserved among the other group-1 NAs. In the two solved N2 structures, which have somewhat atypical sequences, a salt bridge between D147 and H150 appeared to prevent the opening of the 150-loop, despite the presence of V149. Here we test the hypothesis that position 149 is critical for determining the open or closed status of the 150-cavity. Our alternative hypothesis is that cavity status is plastic in the absence of a D147-H150 salt bridge, being dependent on loop conformations that are themselves flexible. Earlier computational studies of N1 from avian H5N1 showed that this isolate exhibited remarkable flexibility in the 150-loop [6] . The same avian N1 was also reported to contain a closed 150-loop under certain crystallization conditions [1] and additionally shown to be able to switch to a closed loop position during a molecular dynamics (MD) simulation initiated from the co-crystallized oseltamivir-bound open-150-loop configuration [6] . The understanding that emerged was that the avian N1 was able to adopt a wide range of configurations in the 150-loop region, favouring an open conformation of the 150-cavity overall. We examined the flexibility of the 150-cavity area in the 09N1 crystal structure through molecular dynamics simulations using 09N1 and other available structures of N1 and N2 alleles derived from human clinical isolates. In combination with the simulations, an extensive bioinformatics analysis for these alleles in the 150- and 430-loop regions offers new clues as to the controlling features of 150-cavity formation in these critical enzymes. Ultimately, we found that a key salt bridge appears to control the 150-cavity formation in both group-1 and group-2 enzymes, both of which are able to adopt flexible loop conformations in this critical region. We propose that this new structural understanding can be related to antiviral design for any of the influenza NA enzymes. Molecular dynamics simulations To probe the effect of sequence on the atomic-level structure and dynamics of these critical enzymes, we performed four separate 100-ns molecular dynamics simulations for four tetrameric NA enzymes: (1) A/California/04/2009, an H1N1 virus isolated early in the 2009 pandemic (09N1, Protein Data Bank (PDB) accession code: 3NSS ) [5] . We note that the N1 allele in the pandemic strain had recently evolved from an Eurasian-lineage H1N1 swine virus [7] . (2) A mutant N1 that we engineered in silico from A/California/04/2009 by substituting Val for Ile at position 149 (09N1_I149V). (3) A/Vietnam/1203/04, an avian-derived H5N1 virus isolated from a human (VN04N1, PDB accession code: 2HTY ) [1] . (4) A/Tokyo/3/67, a seasonal human H2N2 virus (N2, PDB accession code: 1NN2 ) [8] . 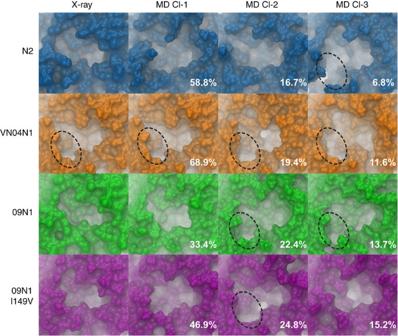Figure 1: Solvent accessible surface area of NA-binding site. The solvent accessible surface area of the NA-binding site is shown, as computed by the MSMS30program, for the X-ray structure, and top three most dominant central member cluster structures (population percentages indicated in white text for each cluster), shown for A/Tokyo/3/67 (N2), A/Vietnam/1203/04 (VN04N1), A/California/04/2009 (09N1) and the 09N1_I149V mutant strain. The open 150-cavity, where present, is outlined with a dotted circle. We note that the I149V mutation in A/Tokyo/3/67 is atypical for a human N2 allele ( Table 1 ; Supplementary Table S1 ). Table 1 Variation in the 150- and 430-loops of N1 and N2 NA alleles of avian, swine and human influenza viruses. Full size table The homotetramer configuration of NA allows us to take advantage of multicopy simulation sampling [9] , amounting to the equivalent of nearly half a microsecond (400 ns) of sampling for each NA monomer, while accounting for realistic neighbouring subunit effects within the structural dynamics. Alpha-carbon root mean square deviation (RMSD) plots for the tetramer systems and individual monomer chains exhibit stability over 100 ns, and there is good agreement between experimental and simulation-derived B-factors ( Supplementary Figs S1–S3 ). Pandemic 2009 H1N1 exhibits open 150-cavity Our simulations reveal that the pandemic 09N1 NA is able to adopt open 150-cavity conformations in normal solution dynamics, and, in contrast to the crystal structure, it appears to favour an open 150-cavity conformation overall ( Fig. 1 ; Table 1 ). In the simulations of 09N1, the 150-loop transitions to an open configuration by 50 ns in all chains of the tetramer ( Supplementary Fig. S4 ). As a reference for open- and closed-loop structures, the PDB accession codes 2HTY and 2HU4 were utilized, respectively. The open 150-cavity crystal structure (2HTY with hydrogen atoms added) exhibits a 150-cavity volume of 36 Å 3 as computed by POVME [10] ( Supplementary Table S3 ). Closed 150-cavity crystal structures (1NN2, 2HU4, 3NSS with hydrogen atoms added) were used as references and uniformly exhibit a volume of 0 Å 3 . To quantify the extent to which structures within the dynamical ensemble adopt either a closed or open 150-cavity conformation, a time series of the pocket volume was computed over the course of the trajectory ( Fig. 2a ; Supplementary Fig. S5 ). Structures were subsequently classified as open or closed based on 150-cavity volume, that is, cavities with volumes greater than or equal to 18 Å 3 , or at least half of the crystal structure open-cavity volume, are considered 'open.' 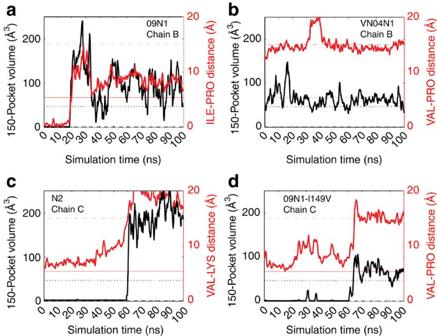Figure 2: Time series analysis of 150-cavity volume and width for a particular monomer in each of the simulated systems. On the left-sideyaxis, the volume of the 150-cavity is computed over the course of simulation. The distance between alpha-carbon of residue 431 (PRO ina,b,d; LYS inc) and the closest side-chain carbon of residue 149 (Val149 panelsb,c,d; ILE ina) is computed and shown in red and the right-sideyaxis. The black and red dotted lines correspond to the open crystal structure (2HTY) volume and distance, respectively; whereas the black dashed and red solid lines correspond to the closed crystal structure (2HU4) volume and distance, respectively. The systems shown are A/Tokyo/3/67 (N2), A/Vietnam/1203/04 (VN04N1), A/California/04/2009 (09N1) and the 09N1_I149V mutant strain. Through this method, we determined that the 09N1 system adopts an open 150-cavity during the majority of the simulation (60.8%, Table 2 ). We note that longer simulation times may further increase the percentage of 09N1 in the open conformation, overcoming the structural bias due to the simulation being initiated with a closed 150-cavity. Figure 1: Solvent accessible surface area of NA-binding site. The solvent accessible surface area of the NA-binding site is shown, as computed by the MSMS [30] program, for the X-ray structure, and top three most dominant central member cluster structures (population percentages indicated in white text for each cluster), shown for A/Tokyo/3/67 (N2), A/Vietnam/1203/04 (VN04N1), A/California/04/2009 (09N1) and the 09N1_I149V mutant strain. The open 150-cavity, where present, is outlined with a dotted circle. Full size image Figure 2: Time series analysis of 150-cavity volume and width for a particular monomer in each of the simulated systems. On the left-side y axis, the volume of the 150-cavity is computed over the course of simulation. The distance between alpha-carbon of residue 431 (PRO in a , b , d ; LYS in c ) and the closest side-chain carbon of residue 149 (Val149 panels b , c , d ; ILE in a ) is computed and shown in red and the right-side y axis. The black and red dotted lines correspond to the open crystal structure (2HTY) volume and distance, respectively; whereas the black dashed and red solid lines correspond to the closed crystal structure (2HU4) volume and distance, respectively. The systems shown are A/Tokyo/3/67 (N2), A/Vietnam/1203/04 (VN04N1), A/California/04/2009 (09N1) and the 09N1_I149V mutant strain. Full size image Table 2 Population analysis based on open or closed 150-cavity. Full size table RMSD-based clustering of the 150-loop residues enables an atomic-level population-based structural analysis. Although the most populated cluster, that is, the cluster that comprises at least 33% of the sampled ensemble, has a closed 150-loop configuration, structures within the next two most populated clusters adopt open 150-cavity configurations ( Fig. 1 ; Supplementary Table S2 ). Figure 2 clearly shows that the second most dominant cluster from the 09N1 simulations has an open 150-loop, highly similar to the open 150-loop of VN04N1. By comparison, the VN04N1 150-cavity is consistently open throughout the simulations, being present for 93.4% of the trajectory ( Figs 1 and 2b ; Table 1 ; Supplementary Fig. S6 ). The formation of a stable and open 150-cavity in 09N1 indicates that the structural dynamics of the recent pandemic strain appear to be more similar to the classic group-1 isolates than to the group-2 isolates, in contrast to what the static crystal structure suggests. This finding provides an atomic-level structural understanding of how antiviral compounds designed to take advantage of contacts in the 150-cavity can be active against both the 2009 H1N1 and 2004 Vietnam H5N1 isolates, as very recently shown in ref. 3 . 150-Cavity formation controlled by a conserved salt bridge The dynamics of the N2 strain reveal that a key salt bridge between conserved residues D147 and H150 controls the formation of the 150-cavity in N2. This ionic contact locks I149 in the space of the 150-cavity ( Fig. 3 ), as suggested in ref. 5 . However, in each chain of the N2 tetramer simulation, this salt bridge intermittently breaks and then reforms; in chain C, at 60 ns the contact is lost again, after which the open 150-cavity forms, and contact to the 430-loop is lost ( Fig. 2c ; Supplementary Fig. S7 ). The loss of the D147-H150 salt bridge allows the 150-loop to move to the open position, even wider than the VN04N1 open 150-loop structure ( Fig. 2 ). RMSD-based clustering of the 150-loop indicates that while both the first and second most dominant configurations remain closed, the third most dominant configuration, representing 6.8% of the trajectory, exhibits an open 150-cavity ( Fig. 1 ). Volumetric calculations of the 150-cavity confirm that the open-cavity conformation is present in 10% of the simulation and has a volume of 284 Å 3 . For the remainder of the simulation, the salt bridge does not reform, and the wide-open 150-cavity therefore persists in one chain of the N2 tetramer. 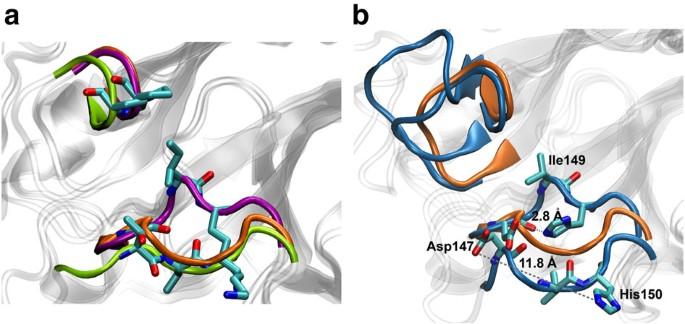Figure 3: Structural variation in N1 and N2 clinical isolates. (a) The 150- and 430-loop structures are shown for 09N1 crystal structure (purple), 09N1 second most dominant molecular dynamics (MD) cluster representative structure (green backbone) and VN04N1 crystal structure (orange), indicating that the pandemic N1 adopts an open 150-loop conformation. Gly147, Ile149, Lys150 and Pro431 are shown in stick representation. (b) N2 150- and 430-loops from crystal and most dominant cluster representative structures are shown in blue, and open VN04N1 crystal structure are shown in orange. The D147-H150 salt bridge spontaneously ruptures in chain C of N2, extending its initial contact from 2.8 Å in crystal structure to 11.8 Å in the most dominant MD-generated cluster structure, revealing a wide-open 150-cavity. Figure 3: Structural variation in N1 and N2 clinical isolates. ( a ) The 150- and 430-loop structures are shown for 09N1 crystal structure (purple), 09N1 second most dominant molecular dynamics (MD) cluster representative structure (green backbone) and VN04N1 crystal structure (orange), indicating that the pandemic N1 adopts an open 150-loop conformation. Gly147, Ile149, Lys150 and Pro431 are shown in stick representation. ( b ) N2 150- and 430-loops from crystal and most dominant cluster representative structures are shown in blue, and open VN04N1 crystal structure are shown in orange. The D147-H150 salt bridge spontaneously ruptures in chain C of N2, extending its initial contact from 2.8 Å in crystal structure to 11.8 Å in the most dominant MD-generated cluster structure, revealing a wide-open 150-cavity. Full size image The spontaneous loss of this key contact under 'physiologically relevant' simulation conditions provides a clear atomic-level model for 150-cavity formation in the N2 clinical isolate. The loss of the salt bridge reduces the rigidity of the 150-loop, enabling the loop to sample more open conformations. Contacts with the neighbouring 430-loop are simultaneously lost, and significant expansions of both the 150- and 430-cavities occur ( Figs 1 , 2C and 3 ; Supplementary Table S3 and Supplementary Fig. S8 ). Although the open 150-loop is energetically accessible in the N2 structures, its low population during the simulation makes it unlikely that this open 150-cavity would appear in X-ray crystallography experiments. Such a cavity would be able to accommodate compounds targeting the 150-cavity, albeit with a lower affinity, as very recently shown in ref. 3 . In all the N1 proteins, D147 is replaced with an uncharged G147, and therefore no salt bridge is present to lock I/V149 in the 150-cavity space. This may explain why an open 150-cavity is characteristically observed in crystals, even in 09N1, which is able to adopt a stable open 150-cavity conformation. It also underscores the importance of considering solution-phase dynamics for these enzymes and not only crystallographic information, which is generally only able to provide one low-energy snapshot of the dynamic protein complex under crystalline conditions. Among N1 alleles for which structures exist, the 2009 H1N1 pandemic isolate uniquely contains an I149. Thus, Li et al . [5] hypothesized that the additional extension of the I149 side chain, compared with V149, may be a compensating factor in controlling the closed-loop structure, despite strict conservation of all other residues in this area. Structurally, the longer side chain of I149 may facilitate van der Waals contacts to the neighbouring 430-loop, and shift the population to a more closed 150-loop state; a V149 mutation would facilitate loss of contact between the 150- and 430-loop, shifting the population to a more open 150-cavity state. To test this hypothesis, we created the 09N1_I149V mutant strain in silico and performed an identical 100 ns simulation. Our results indicate that the effect of this mutation on 150-cavity status varies due to 150-loop flexibility. The time series data indicate that the I149V mutation caused chain D to open almost immediately, chain C to open after 60 ns, chain A to open intermittently and had almost no effect on chain B ( Supplementary Fig. S9 ). Overall, the 09N1_I149V mutant is actually more closed, exhibiting the open 150-cavity less frequently, in only 37.1% of the simulation, compared with the normal 09N1 strain with the I149 present ( Table 2 , Fig. 2d ; Supplementary Fig. S9 ). Moreover, only one of the three most dominant structures, cluster 2, presents the open 150-cavity, and thus, the V149 by itself cannot explain the behaviour of the 09N1_I149V. Analysis of sequence conservation in the 150-loop region To date, the evolutionary distribution of the 150-cavity among NA alleles has been inferred primarily from crystallographically resolved structures, which represent a limited subset of the genetic variation of NAs in nature. Based on those analyses, it seemed logical to attribute the occurrence of an open 150-cavity to having a V or I at position 149, and by extension, to membership, in the group-1 or group-2 NAs, respectively, as shown in figure 3 of Li et al . Our dynamical analyses suggest that I/V149 is not as critical to 150-cavity status as the D147-H150 salt bridge, which warrants re-examination of the association of cavity status with NA group membership. We determined the distribution of genetic variation in the 150 and 450 loops among all avian, human and swine N1 and N2 sequences that had been deposited in GenBank and Global Initiative on Sharing Avian Influenza Data (GISAID) as of 12 August 2010 using phylogenetic analysis to construct consensus sequences for each major clade ( Supplementary Methods for methodological details). Our phylogenetic analyses ( Table 1 ) show that no single amino acid position in the 150- or 430-loops clearly differentiates the N1 and N2 alleles, which are in group-1 and group-2, respectively. The D147-H150 salt bridge is not a defining characteristic of N2 alleles, as it is not present in avian viruses, which were the source of the N2 allele in the 1957 H2N2 human pandemic strain. Nor is the salt bridge found in human H3N2 viruses that have been circulating since 2008, due to fixation of a D147N mutation. Thus, neither the amino acid at position 149 nor the salt bridge is fixed characters that differentiate group 1 and group 2 NAs. Nor do they, at least by themselves, characterize viruses capable of infection of humans. Additional tests of our hypothesis require the acquisition of crystal structures of additional NA alleles, most critically, an N2 allele that contains both the D147-H150 salt bridge and I149. Our results highlight the importance of interpreting influenza NA sequence and structural data in light of the dynamical ensemble of conformations that are accessible to each NA protein. This work shows for the first time that both N1 and N2 clinical isolates exhibit flexibility in the 150-cavity neighbouring the conserved sialic-acid-binding site. Although it remains possible that the open and closed conformation observed in crystal structures may be due to differences in crystallization conditions or procedures, our results indicate that the presence of the 150-cavity is not a strictly defining characteristic for group-1 or group-2 NA enzymes. Instead, it appears that both N1 and N2 enzymes are able to adopt an open 150-cavity within their solution phase structural ensemble, in various relative populations, which appear to be predominantly controlled by the presence of the D147-H/R150 salt bridge. This suggests a new paradigm for the understanding of the presence of the 150-cavity in both group-1 and group-2 NAs. The inherent flexibility of the 150- and 430-loops may have a role in full glycan receptor recognition, and in particular, with facilitating recognition events with the distal sugar residues of different glycan receptors. It is likely that the opening and closing of the 150-cavity is required for natural sialoglycan substrates to fit into the active site, given the bulky nature of these glycans. This study additionally underscores the need to consider dynamics in rationalizing the structure–function relationships of various antiviral–NA pairs. Ensemble-based drug discovery approaches [11] that account for full-receptor flexibility towards NAs that do not contain the D147-H150 salt bridge will likely present additional advances in the design of compounds that selectively target the 150-cavity, opening the possibility for receptor-specific inhibitors. In closing, we note that whether the flexibility of the NA-binding site has an impact on receptor specificity, virus transmissibility or pathogenicity remains to be seen and will likely require a better understanding of HA receptor-binding domain dynamics for each of the NA/HA pairs found in humans [12] . Simulation protocol System setup was performed as follows for all simulated systems. Atomic coordinates were taken from 2HTY for A/Vietnam/1203/04 (VN04N1) [1] , 3NSS for A/California/04/2009 (09N1) [5] and 1NN2 for A/Aichi/3/67 (N2) [8] . Protonation states for histidines and other titratable groups were determined at pH 6.5 by the PDB2PQR [13] web server using PROPKA [14] and manually verified. All crystallographically resolved water molecules and calcium ions were retained where possible and taken by homology from 2HTY if not present. The system was setup using the AMBER11 [15] program xLeap using the AMBER99SB force field [16] . Disulphide bonds were properly enforced using the CYX notation in AMBER. A 10–12 Å pad of TIP3P waters was added to solvate to each system. Neutralizing counter ions were added to each system. In order to mimic experimental assay conditions, a 20 mM NaCl salt bath was introduced. System details and additional methodological information can be found in the Supplementary information . N1 and N2 tetramer simulations were performed with a version of the PMEMD module from AMBER 11 that was custom tuned for these specific simulations and the NICS Cray XT4 and SDSC Trestles supercomputers by SDSC under the NSF's TeraGrid Advanced User Support Program. The N1 and N2 apo tetramer complexes were minimized and equilibrated as follows: in order to alleciate any steric clashes before performing molecular dynamics, the structures were minimized in a number of stages in which harmonic restraints of initially 5 kcal mol −1 Å −2 on all non-hydrogen protein atoms were slowly reduced over ~40,000 combined steepest descent and conjugate gradient minimization steps. Following minimization, the system was linearly heated to 310 K in the canonical NVT ensemble (constant number of particles, N; constant volume, V; constant temperature, T) using a Langevin thermostat, with a collision frequency of 5.0 ps −1 , and harmonic restraints of 4 kcal mol −1 Å −2 on the backbone atoms. Then, a further three 250 ps long runs at 310 K were conducted in the NPT ensemble with the restraint force constant being reduced by 1 kcal mol −1 Å −2 each time and pressure controlled using a Berendsen barostat [17] with a coupling constant of 1 ps and a target pressure of 1 atm. A final 250 ps of NPT dynamics was run at 310 K without restraints and a Langevin collision frequency of 2 ps −1 . Production runs were then made for 100 ns duration in the NVT ensemble at 310 K. As with the heating, the temperature was controlled with a Langevin thermostat (but with a 1.0 ps −1 collision frequency). The time step used for all stages was 2 fs and all hydrogen atoms were constrained using the SHAKE algorithm [18] . Long-range electrostatics were included on every step using the Particle Mesh Ewald algorithm [19] with a 4th order B-spline interpolation, a grid spacing of <1.0 Å, and a direct space cutoff of 8 Å. For all trajectories, the random number stream was seeded using the wall clock time in microseconds. The production trajectories for each monomer of the tetramer were extracted and concatenated to approximate 400 ns of monomer sampling. RMSD clustering RMSD clustering was performed as implemented in the rmsdmat2 and cluster2 programs of the GROMOS++ analysis software [20] . A total of 500 tetramer structures were collected by sampling at 200 ps intervals. Monomer structures were then concatenated together, yielding a total of 2,000 structures. Before clustering, external translational and rotational motions were removed by minimizing the RMSD distance of the alpha-carbon atoms of the sampled structure to the equivalent atoms of the first frame of chain A. Using a 2.6 Å cutoff, clustering was then performed using the GROMOS++ clustering algorithm [21] in Gromacs [22] on the alpha-carbon atoms of the 6-residue subset, 146–152, which comprise the 150 loops. Each cluster contains a central structure, or 'cluster representative member,' called the 'centroid,' whose RMSD is equidistant to all other cluster members. The cluster representative's structural properties are considered characteristic of all cluster members. Cluster results are summarized in Table 2 . RMSD and B-factor calculations B-factor calculations, as well as tetramer and monomer RMSD time series, were performed using the ptraj analysis tool in the AMBER 10 program suite [23] . Structures were sampled at 20 ps intervals. Before performing each calculation, external translational and rotational motions were removed by minimizing the RMSD distance of the alpha-carbon atoms to the equivalent atoms of the first frame of the trajectory. RMSD and B-factor values were calculated for alpha-carbon atoms. 09N1 RMSD 150-loop measurements RMSD values were measured using a custom, hand-written script in the VMD TCL-TK console [24] . Structures were sampled at 20 ps intervals. Sampled structures of each monomer were RMSD-aligned by alpha-carbon to the equivalent alpha-carbon atoms of the 'reference' structure: chain A of PDB ID 2HTY, open reference; or chain A of PDB ID 2HU4, closed reference. Following alignment, the RMSD of the 150 loop of each monomer was measured with respect to the 150 loop of each reference structure. The 150 loops were defined as residues 146–152 for the 09N1 monomers, as well as for the open and closed reference structures. Interatomic distance measurements The distance separating the salt bridge pair ASP147 and HIS150 was measured using a custom, hand-written script in the VMD TCL-TK console. Structures were sampled at 20 ps intervals. The distance between the two residues was defined as the distance separating centres of mass of the heavy atoms of the ASP147 carboxylate and the HIS 150 imidazole. The distance between residues 149 and 431 were measured for each step using a custom VMD script. Neuraminidase volume population analysis The numbers of open or closed 150-cavity conformations out of a total of 2,000 snapshots were computed. Any instantaneous volume equal to or greater than half the volume of the crystal structure of canonical group-1 serovar (2HTY exhibits a total 150-cavity volume of 36 Å 3 ) is considered to be 'open'. Otherwise the 150-cavity is considered 'closed' (that is, when it exhibits <18 Å 3 ). The volume of the 150-cavity was measured for each step by using POVME [10] ; a pocket volume measuring algorithm. To measure the volume, we used a single inclusion sphere that encompassed the 150-cavity. The POVME algorithm neglected the volume occupied by NA atoms and not spatially contiguous with a point specified within the 150-cavity. By rotating 90° around the NA tetramer central axis, each of the other three 150-cavity sites were specified. The volume was thus measured for every snapshot of the simulation on all four chains of each NA. Figures and plots Matlab was used to generate all plots and molecular images were created using VMD [24] . Consensus sequences We downloaded all influenza A N1 and N2 gene sequences from humans, avians and swine that were >600 bp in length from GenBank and GISAID on 12 August 2010. We aligned sequences using ClustalX 2.0 (ref. 25 ) and constructed phylogenetic trees using MrBayes version 3.1.2 (ref. 26 ) using the GTR+I+gamma model, as suggested by jmodeltest version 0.1.1 (ref. 27 ) under the Akaike Information Criterion. All other MrBayes parameters were set to the default. We allowed MrBayes to run, sampling every 1,000 trees, until the Monte Carlo Markov chains converged as determined by Tracer software version 1.5 (ref. 28 ). We discarded the burn-in as determined by Tracer. Similar results were obtained using the neighbour-joining routine of PAUP* 4.0b10 (ref. 29 ; results not shown). Consensus sequences containing amino acids found at a frequency of at least 80% were constructed for each major evolutionary clade. Results are shown, along with samples sizes, in Table 1 . How to cite this article: Amaro, R. E. et al . Mechanism of 150-cavity formation in influenza neuraminidase. Nat. Commun. 2:388 doi: 10.1038/ncomms1390 (2011).